Femtolitre chemistry assisted by microfluidic pen lithography Chemical reactions at ultrasmall volumes are becoming increasingly necessary to study biological processes, to synthesize homogenous nanostructures and to perform high-throughput assays and combinatorial screening. Here we show that a femtolitre reaction can be realized on a surface by handling and mixing femtolitre volumes of reagents using a microfluidic stylus. This method, named microfluidic pen lithography, allows mixing reagents in isolated femtolitre droplets that can be used as reactors to conduct independent reactions and crystallization processes. This strategy overcomes the high-throughput limitations of vesicles and micelles and obviates the usually costly step of fabricating microdevices and wells. We anticipate that this process enables performing distinct reactions (acid-base, enzymatic recognition and metal-organic framework synthesis), creating multiplexed nanoscale metal-organic framework arrays, and screening combinatorial reactions to evaluate the crystallization of novel peptide-based materials. Chemical reactions at volumes from femtolitres (10 −15 litres) to attolitres (10 −18 litres) are becoming increasingly necessary to study biological processes that occur in small volumes of cellular compartments [1] , [2] , [3] , [4] and liquid-phase reactions [5] , to synthesize homogenous nanostructures [6] and to perform high-throughput assays and combinatorial screening [7] , [8] . To perform reactions on surfaces and at such dimensions, it is critical to manipulate and confine ultrasmall volumes of reagents and control their mixing into well-defined compartments. It is also important to control the dimensions and monodispersity of these reactors, their positioning to facilitate monitoring and the evaporation rate of all solvents used. To date, methods to conduct reactions at these ultrasmall dimensions can be classified into two types based on the use of micromachining techniques (mainly microfluidics and femtolitre wells [9] , [10] , [11] , [12] ) and self-enclosed volume elements, including vesicles, micelles and oil/water-dispersed droplets [13] , [14] , [15] , [16] , [17] , [18] . We propose here an alternative approach to realize femtolitre reactions on a surface by handling and mixing femtolitre volumes of reagents using a microfluidic stylus. This approach, named microfluidic pen lithography (MPL), overcomes the high-throughput limitations of vesicles and micelles and obviates the usually costly step of fabricating microdevices and wells: it can be employed to mix reagents in isolated femtolitre droplets that can be used as reactors to conduct independent reactions and/or crystallization processes over centimetre-scale regions with high registration accuracy. In particular, we have found that conventional pen lithography technologies and tools [19] , [20] , [21] , [22] , commonly used for molecular and material printing, and now available to many researchers, are ideal for running such reactions on surfaces. Microfluidic pens (BioForce, USA; see Supplementary Fig. S1 ) offer high levels of uniformity and reproducibility for depositing femtolitre volumes of liquids onto surfaces. Dip-Pen Nanolithography [19] NLP-2000 platform (NanoInk Inc., USA), equipped with a five-axis stage system and commercial lithography software, guarantees the control of the dwell time and the vertical and translational motion of the surface relative to the microfluidic pens (±75 nm z precision and ±100 nm positional precision over areas as large as 16 cm 2 ). This high accuracy enables the programmable positioning of microfluidic pens on top of selected, pre-patterned femtolitre droplets, followed by their precise approach up to the surface contact area. This straightforward MPL method comprises two steps: femtolitre droplet generation, and femtolitre volume delivery into these droplets ( Fig. 1a ; also see Supplementary Movie 1 ). It enables mixture of femtolitre volumes containing reagents directly on surfaces, thus forming well-defined mixture droplets in which individual femtolitre reactions can be conducted. Finally, an environmental humidity chamber included in the lithographic platform enables such reactions to be run under controlled atmospheres (that is, humidity or organic solvent vapour levels) and reduces droplet evaporation. This latter factor is crucial, as the second reagent must be delivered into the patterned droplets before they evaporate, and the resulting mixture droplet requires sufficient time to react and crystallize. Droplet evaporation can be also minimized by using reagent solutions containing high-boiling point, low-volatility solvents that do not affect the desired reaction. In this study, we demonstrate that MPL enables performing distinct reactions (acid-base, enzymatic recognition and metal-organic framework (MOF) synthesis), creating multiplexed nanoscale MOF arrays, and screening combinatorial reactions to evaluate the crystallization of novel peptide-based materials. We believe that this method could be adopted by researchers as a desktop tool to synthesize and crystallize nanomaterials at desired locations, fabricate arrays and devices, perform combinatorial screening and/or study reactions at the femtolitre scale. 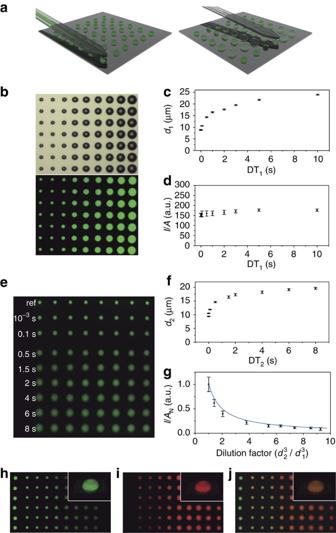Figure 1: Femtolitre delivery and mixing capabilities of MPL. (a) Schematic illustration of the two-step MPL method, showing the patterning of an array of SoF droplets (step 1), followed by precise delivery of different volumes of a solution into them (step 2). (b) Bright-field optical and corresponding confocal fluorescence microscopy images (λexc=488 nm;λem=500–575 nm) of an array of SoF droplets (droplet distance=28 μm) created by using different DT1. (c,d) DT1dependence ofd1and ofI/Ameasured for each droplet series. (e) Confocal fluorescence microscopy image of an array of SoF droplets (droplet distance=35 μm), in which femtolitre volumes of an H2O/glycerol solution were added at different DT2. Note that the top row corresponds to bare SoF droplets. (f) DT2dependence of d2. (g) Dilution factor dependence ofI/AN. The line represents the expected behaviour of a bulk SoF solution (assuming that the decrease in fluorescence intensity is due only to dilution). (h–j) Confocal fluorescence microscopy images (λexc=488 nm;λem=500–575 nm (h);λexc=633 nm;λem=600–785 nm (i); and superimposed previous images (j)) of an array of SoF droplets (droplet separation=28 μm), in which femtolitre volumes of a solution of Nile Blue were added at different DT2. Note that the left and right columns correspond to pure SoF and Nile Blue droplets, respectively, whereas the gradient of colours from yellow/orange to red (left to right) denotes the increase in concentration of Nile Blue relative to SoF. In (c,d,f,g) the error bars represent the s.d. of the average results obtained for all equivalent droplets in the array. Figure 1: Femtolitre delivery and mixing capabilities of MPL. ( a ) Schematic illustration of the two-step MPL method, showing the patterning of an array of SoF droplets (step 1), followed by precise delivery of different volumes of a solution into them (step 2). ( b ) Bright-field optical and corresponding confocal fluorescence microscopy images ( λ exc =488 nm; λ em =500–575 nm) of an array of SoF droplets (droplet distance=28 μm) created by using different DT 1 . ( c , d ) DT 1 dependence of d 1 and of I / A measured for each droplet series. ( e ) Confocal fluorescence microscopy image of an array of SoF droplets (droplet distance=35 μm), in which femtolitre volumes of an H 2 O/glycerol solution were added at different DT 2 . Note that the top row corresponds to bare SoF droplets. ( f ) DT 2 dependence of d 2 . ( g ) Dilution factor dependence of I / A N . The line represents the expected behaviour of a bulk SoF solution (assuming that the decrease in fluorescence intensity is due only to dilution). ( h – j ) Confocal fluorescence microscopy images ( λ exc =488 nm; λ em =500–575 nm ( h ); λ exc =633 nm; λ em =600–785 nm ( i ); and superimposed previous images ( j )) of an array of SoF droplets (droplet separation=28 μm), in which femtolitre volumes of a solution of Nile Blue were added at different DT 2 . Note that the left and right columns correspond to pure SoF and Nile Blue droplets, respectively, whereas the gradient of colours from yellow/orange to red (left to right) denotes the increase in concentration of Nile Blue relative to SoF. In ( c , d , f , g ) the error bars represent the s.d. of the average results obtained for all equivalent droplets in the array. Full size image Patterning and mixing capabilities at the femtolitre scale We evaluated the first step of this method—including, creation of femtolitre droplet arrays, reproducibility and homogenous volume and reagent delivery—through delivery of a sodium fluorescein (SoF) solution onto a SiO 2 surface. In a typical experiment, the microfluidic pen was first loaded with a dimethylsulphoxide (DMSO)/glycerol (1:1) solution of SoF, mounted onto the lithographic platform at an acute angle of 10°, and used to fabricate an array of droplets by bringing it into contact with the surface for 0.001–10 s (hereafter, DT 1 : dwell time used in step 1) at 60% relative humidity (RH; Fig. 1b ; also see Supplementary Fig. S2 for a three-dimensional reconstruction of the droplet array). The patterned green fluorescent droplets had diameters ( d 1 ) from 8.8±0.2 to 24.0±0.2 μm ( Fig. 1c ), confirming that DT 1 can be used to control the size (and therefore the estimated volumes, which vary from 42.7±2.3 to 873.4±20.9 fL, considering a measured macroscopic contact angle of 34.6±0.3°; see also Supplementary Methods ) of the initial droplets patterned by MPL. To demonstrate homogeneous concentration delivery, we measured the average of the fluorescence mean intensity per surface area ( I / A —as a measure of dye concentration in the droplets, we analysed the fluorescence image slice corresponding to the droplet volume in direct contact with the surface, summed the intensity values for all fluorescent pixels of the droplet, and then divided by the droplet area in that image; also see Supplementary Methods ) for each droplet series patterned at a different DT 1 . Significantly, we observed <6% deviation in I / A among the droplet series ( Fig. 1d ). To demonstrate the ability of controlling the deposition of a second femtolitre volume on top of the pre-patterned droplets (step 2), we delivered femtolitre volumes of an H 2 O/glycerol (1:1) mixture into pre-patterned H 2 O/glycerol (1:1) droplets of SoF ( d 1 =9.4±0.1 μm). The H 2 O/glycerol solution was delivered at dwell times (hereafter DT 2 : dwell time used in step 2) of 0.001 to 8 s at 50% RH, forming an array of mixture droplets with diameters ( d 2 ) from 10.5±0.1 to 19.7±0.4 μm, respectively ( Fig. 1e ). Figure 1f shows that the delivered volume increased with increasing DT 2 . Based on this finding, we concluded that DT 2 could be used to control the volume delivered into the pre-patterned droplets and, therefore, to control the concentration of SoF in each mixture droplet. This is demonstrated in Fig. 1g and Supplementary Fig. S3 , in which the average I / A measured for each droplet series normalized to the average of the I / A measured for the initial SoF concentration ( I / A N ) is plotted as a function of the dilution factor ( V 2 / V 1 = d 2 3 / d 1 3 ) and of DT 2 . When DT 2 is increased, the SoF concentration in each mixture droplet—and consequently, I / A N —decreases according to the volumes of H 2 O/glycerol added, following the expected behaviour of a bulk SoF solution (assuming that the decrease in fluorescence intensity is due only to dilution). This dependence was reproducibly obtained (see Supplementary Fig. S4 ), demonstrating that DT 2 can effectively be used to control the ratio of reagents in the mixture droplets. Another factor contributing to this ratio is cross-contamination, which can affect the homogeneous mixing between mixture droplets. The influence of this phenomenon was evaluated by analysing the I / A of several droplets patterned at DT of 2 s after delivering an H 2 O/glycerol (1:1) mixture into pre-patterned H 2 O/glycerol (1:1) droplets of SoF ( d 1 =8.7±0.2 μm) at DT 2 of 0.001–10 s at 45% RH (see Supplementary Fig. S5 ). I / A was detected in the first three droplets for all cases: the average intensity values (relative to the initial SoF intensity) were ca. 6.0% (1st droplet), 2.8% (2nd droplet) and 1.2% (3rd droplet). Based on these values, we decided to introduce a cleaning step to prevent cross-contamination and ensure unadulterated reagent mixing. In the cleaning step, a few droplets are patterned outside the working area (that is, on a different surface) between each round of reagent delivery on top of the pre-patterned droplets. To further verify the delivery capabilities of MPL and homogeneous mixing of the solutions in each mixture droplet, we also delivered a solution of the red-fluorescent dye Nile Blue at different DT 2 into pre-patterned green-fluorescent SoF droplets, and then visualized their fluorescence signal co-localization ( Fig. 1h–j ). 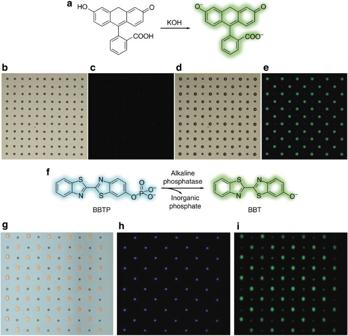Figure 2: MPL-assisted femtolitre reactions. (a) The acid/base reaction between fluorescein acid and KOH. (b,c) Bright-field optical and fluorescence microscopy (λexc=450–490 nm;λem>515 nm) images of an array of fluorescein acid droplets (droplet distance=22 μm) before KOH addition, showing the absence of green fluorescence. (d,e) Bright-field optical and fluorescence microscopy images of the corresponding array after KOH addition, showing aca.Thirty-fold increase in green fluorescence at all alternating mixture droplets. (f) Scheme of the detection of calf intestinal AP enzyme. (g) Bright-field optical image of an array of BBTP droplets (droplet distance=30 μm), in which femtolitre volumes of AP were mixed into alternated droplets. (h) Fluorescence microscopy image of the corresponding array upon UV excitation (λexc=359–371 nm;λem>397 nm), showing the characteristic blue fluorescence of BBTP. (i) Fluorescence microscopy image of the corresponding array upon blue-light excitation (λexc=450–490 nm;λem>515 nm), showing the characteristic green fluorescence of BBT at all mixture droplets arising from AP-catalysed dephosphorylation of BBTP. Acid-base and enzymatic recognition reactions Figure 2a–i show two chemical reactions performed at the femtolitre scale: an acid/base reaction between the non-fluorescent fluorescein acid and its fluorescent dianionic state ( Fig. 2a ), and a biologically-relevant reaction based on the detection of calf intestinal alkaline phosphatase (AP) enzyme ( Fig. 2f ). For the acid/base reaction, we delivered a H 2 O/glycerol (7:3) solution of KOH into alternated pre-patterned DMSO/glycerol (7:3) droplets of fluorescein acid at 50% RH ( Fig. 2b ). Before the KOH delivery ( Fig. 2c ), low fluorescence was detected from all fluorescein droplets, but in the droplets in which KOH was mixed, a ca. 30-fold increase in green fluorescence (corresponding to the deprotonation of fluorescein) was observed ( Fig. 2e ). Note that numerous femtolitre reactions (400 replicas over 0.78 mm 2 area) were successfully run without the microfluidic pens having to be reloaded ( Supplementary Fig. S6 ). Femtolitre reactions of the AP-detection reaction also were performed with a high level of reproducibility. To detect this enzyme through the dephosphorylation of blue fluorescent 2′-[2-benzothiazoyl]-6′-hydroxybenzothiazole phosphate (BBTP) to green fluorescent 2′-[2-benzothiazoyl]-6′-hydroxybenzothiazole (BBT), a diethanolamine (DEA)/glycerol (7:3) droplet array of BBTP was created, and then femtolitre volumes of a DEA/glycerol (7:3) solution of AP were added to alternating droplets in the array at 80% RH ( Fig. 2g ). After the two reagents were mixed, the substrate was incubated at 37 °C and 80% RH for 15 min. The resulting array was first excited at 355 nm: all the BBTP droplets fluoresced blue, whereas none of the mixture droplets fluoresced ( Fig. 2h ). In contrast, when excited at 488 nm ( Fig. 2i ) all the mixture droplets fluoresced green (even though they were more dilute), at approximately twice the intensity of the BBTP droplets. These observations confirmed the proper detection of AP through the complete dephosphorylation of BBTP, thus demonstrating the utility of the MPL method for studying biological reactions at the femtolitre scale. Figure 2: MPL-assisted femtolitre reactions. ( a ) The acid/base reaction between fluorescein acid and KOH. ( b , c ) Bright-field optical and fluorescence microscopy ( λ exc =450–490 nm; λ em >515 nm) images of an array of fluorescein acid droplets (droplet distance=22 μm) before KOH addition, showing the absence of green fluorescence. ( d , e ) Bright-field optical and fluorescence microscopy images of the corresponding array after KOH addition, showing a ca. Thirty-fold increase in green fluorescence at all alternating mixture droplets. ( f ) Scheme of the detection of calf intestinal AP enzyme. ( g ) Bright-field optical image of an array of BBTP droplets (droplet distance=30 μm), in which femtolitre volumes of AP were mixed into alternated droplets. ( h ) Fluorescence microscopy image of the corresponding array upon UV excitation ( λ exc =359–371 nm; λ em >397 nm), showing the characteristic blue fluorescence of BBTP. ( i ) Fluorescence microscopy image of the corresponding array upon blue-light excitation ( λ exc =450–490 nm; λ em >515 nm), showing the characteristic green fluorescence of BBT at all mixture droplets arising from AP-catalysed dephosphorylation of BBTP. Full size image Femtolitre crystallization of MOFs We then evaluated the MLP method for creating well-defined mixture droplets and subsequently using them to confine the synthesis and crystallization of materials (rather than liquid reactions) on surfaces. As proof-of-concept, we reproducibly compartmentalized the crystallization of the archetypical MOF HKUST-1 (ref. 23 ) by mixing femtolitre volumes of two DMSO solutions of Cu(NO 3 ) 2 ·2.5(H 2 O) and trimesic acid on a SiO 2 surface, and placing the resulting mixture droplet array in ambient conditions for 2 h ( Fig. 3a–c ). To increase the complexity and prove that this MPL method can be used to confine the synthesis of different materials into side-by-side mixture droplets in the same array, we created a multiplexed array of crystalline porous Prussian blue analogues (PBAs) [24] , [25] . We selected four PBAs with the general formula M 3 [Co(CN) 6 ] 2 , where M is Cd(II), Zn(II) and Mn(II), and Ag 3 [Co(CN) 6 ]. The multiplexed array was made by first creating a 4 × 4 droplet array of an H 2 O/glycerol (7.5:2.5) solution of K 3 Co(CN) 6 either on SiO 2 or transmission electron microscopy-grid surfaces. Four different microfluidic pens, each one loaded with a different H 2 O/glycerol (7.5:2.5) metal nitrate solution, were used to deliver femtolitre volumes of each metal salt into four selected droplets comprising the array, as shown in Fig. 3d . Mixing of the two solutions into each one of the mixture droplets enabled the immediate formation of nanocrystals corresponding to the four desired PBAs ( Fig. 3e ), as confirmed by the positive matching between the interplanar distances extracted from electron diffraction patterns measured for each synthesized PBAs and the corresponding literature values ( Fig. 3f–i ). 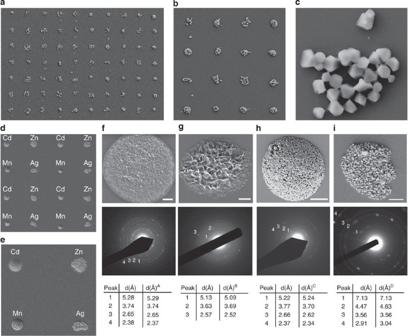Figure 3: Femtolitre synthesis and controlled crystallization of MOFs. (a–c) FESEM images of the synthesized HKUST-1 crystal array (feature distance=25 μm), confirming the reproducibility of the femtolitre droplet-by-droplet reaction and showing the well-defined octahedral shape of the resulting HKUST-1 crystals. (d,e) FESEM images of the multiplexed 4 × 4 array of crystalline PBAs with general formula M3[Co(CN)6]2, where M is Cd(II), Zn(II) and Mn(II), and Ag3[Co(CN)6] (PBA feature distance=25 μm). (f–i) FESEM image of an individual island containing the synthesised Cd(II)-PBA (f), Zn(II)-PBA (g), Mn(II)-PBA (h), Ag(I)-PBA (i) nanocrystals (scale bars, 2 μm), and their corresponding electron diffraction patterns, plus tables comparing the measured interplanar distances (d) with the corresponding literature values: A, JCPDS No. 89-3740; B, JCPDS No. 32-1468; C, JCPDS No. 89–3735; and D, ICSD- 28501. Figure 3: Femtolitre synthesis and controlled crystallization of MOFs. ( a – c ) FESEM images of the synthesized HKUST-1 crystal array (feature distance=25 μm), confirming the reproducibility of the femtolitre droplet-by-droplet reaction and showing the well-defined octahedral shape of the resulting HKUST-1 crystals. ( d , e ) FESEM images of the multiplexed 4 × 4 array of crystalline PBAs with general formula M 3 [Co(CN) 6 ] 2 , where M is Cd(II), Zn(II) and Mn(II), and Ag 3 [Co(CN) 6 ] (PBA feature distance=25 μm). ( f – i ) FESEM image of an individual island containing the synthesised Cd(II)-PBA ( f ), Zn(II)-PBA ( g ), Mn(II)-PBA ( h ), Ag(I)-PBA ( i ) nanocrystals (scale bars, 2 μm), and their corresponding electron diffraction patterns, plus tables comparing the measured interplanar distances (d) with the corresponding literature values: A, JCPDS No. 89-3740; B, JCPDS No. 32-1468; C, JCPDS No. 89–3735; and D, ICSD- 28501. Full size image Screening new metal-peptide networks Finally, as a first proof-of-concept, we tested our method to discover new metal-peptide networks [26] incorporating a randomly selected peptide ligand, glycine-histidine (GH). 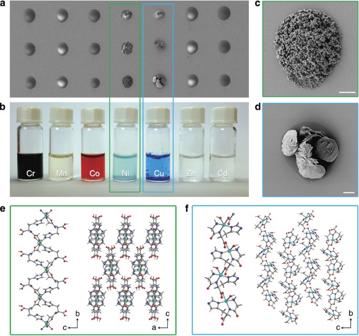Figure 4: Formation and crystallization of peptide-based coordination networks using MLP. (a) FESEM image of a 3 × 7 droplet array in which each row comprises droplets of a mixture containing the GH ligand and one of seven metal acetates (droplet distance=25 μm). Mixture droplets within each row were created by first patterning a droplet of an aqueous solution of 1 M GH (contact time=1 s), and then delivering a solution of the corresponding metal acetate (0.3 M in 7:3 H2O/diethyleneglycol) for different contact times per row: 0.2 s (top), 0.1 s (middle) and 0.01 s (bottom). (b) Photograph showing the bulk reproduction of all screened GH-metal acetate reactions, revealing that the occurrence of crystal formation matched perfectly to the corresponding femtolitre reactions. (c,d) Representative FESEM images of crystals obtained within the femtolitre mixture of Ni(II) (c) and Cu(II) (d) with GH dipeptide. Scale bars: 2 μm. (e,f) X-ray crystal structures of the new [Ni(GH)2]·7H2O and [Cu(GH)(H2O)]·H2O. Figure 4a shows a 3 × 7 combinatorial array of droplets in which we mixed different femtolitre volumes of an aqueous solution of GH with H 2 O/diethyleneglycol (7:3) solutions of various metal acetates (the metals were, from left to right, Cr(III), Mn(II), Co(II), Ni(II), Cu(II), Zn(II) and Cd(II)) at 85% RH. After 2 h of reaction at room temperature, only the droplets corresponding to Ni(II)-GH and Cu(II)-GH mixtures showed the formation of crystals that were stable after cleaning with water ( Fig. 4c ). These screening results were confirmed by reproducing all these reactions in bulk ( Fig. 4b ), from which two [Cu(GH)(H 2 O)]·H 2 O and [Ni(GH) 2 ]·7H 2 O networks were discovered after solving their crystal structures ( Fig. 4e ; also see Supplementary Figs S7–S10 and Supplementary Tables S1–S5 ). Thus, this MPL approach, once enhanced to enable greater control over reaction conditions such as temperature, will likely have important applications in biology, chemistry and materials science. Furthermore, it will be ideal for fabricating arrays of complex structures that can only be prepared via chemical synthesis (for example, crystals), thus making it potentially useful for electronics and sensors. Figure 4: Formation and crystallization of peptide-based coordination networks using MLP. ( a ) FESEM image of a 3 × 7 droplet array in which each row comprises droplets of a mixture containing the GH ligand and one of seven metal acetates (droplet distance=25 μm). Mixture droplets within each row were created by first patterning a droplet of an aqueous solution of 1 M GH (contact time=1 s), and then delivering a solution of the corresponding metal acetate (0.3 M in 7:3 H 2 O/diethyleneglycol) for different contact times per row: 0.2 s (top), 0.1 s (middle) and 0.01 s (bottom). ( b ) Photograph showing the bulk reproduction of all screened GH-metal acetate reactions, revealing that the occurrence of crystal formation matched perfectly to the corresponding femtolitre reactions. ( c , d ) Representative FESEM images of crystals obtained within the femtolitre mixture of Ni(II) ( c ) and Cu(II) ( d ) with GH dipeptide. Scale bars: 2 μm. ( e , f ) X-ray crystal structures of the new [Ni(GH) 2 ]·7H 2 O and [Cu(GH)(H 2 O)]·H 2 O. Full size image We have reported a new, highly versatile lithographic method, MPL, for doing femtolitre chemistry on surfaces by handling and mixing femtolitre volumes of reagents. Albeit this nascent form of MPL includes only a microfluidic single pen, it can reproducibly perform a broad range of femtolitre reactions in water and organic solvents, and enables the confined crystallization of nanomaterials at precise locations on surfaces in a spatially ordered and combinatorial manner. We are confident that MPL could be greatly enhanced in scope and capability through the introduction of microfluidic multi-pens, analogously to the evolution recently undergone by other nanolithography methods that began with a single pen (for example Dip-Pen Nanolithography). Furthermore, method development to optimize crucial reaction parameters (for example, humidity, temperature, surface type, evaporation rate, possible cross-contamination and so on), should provide access to an ever widening scope of femtolitre reactions and crystallizations on diverse surfaces. Finally, we are cautiously optimistic that as MPL matures and becomes more sophisticated, it will ultimately enable researchers to run high-throughput assays and combinatorial screening, perform femtolitre-scale biological studies, and even discover novel materials based on expensive building blocks. Substrate preparation and microfluidic pen lithography Si/SiO 2 substrates were subsequently sonicated for 10 min. in acetonitrile, ethanol and MilliQ water, and dried with N 2 gas flow. Each microfluidic pen was cleaned in piranha solution (3:1 v/v solution of H 2 SO 4 and 30% H 2 O 2 ) for 20 min., rinsed with MilliQ water and dried with slight N 2 gas flow. Caution: piranha solution is a strong acid and oxidant and should be handled with extreme care. Afterwards, each pen was introduced in an UV/ozone chamber for 20 min., and was then loaded with the corresponding reagent solutions by adding 1.5 μl of the appropriate solutions into the reservoir via micropipette. MPL-assisted femtolitre reactions were run on an NLP-2000 Nanolithography Platform at room temperature and at relative humidities of 50–85%. Array of SoF droplets delivered at different DT 1 An array of 7 × 9 droplets (droplet separation=28 μm) of 0.01 M SoF (in DMSO/glycerol, 1:1 v/v) was patterned on a SiO 2 surface at DT 1 =0.001, 0.01, 0.1, 0.5, 1, 2, 3, 5 and 10 s at room temperature under a RH of 60%. Mixture droplet arrays An array of 8 × 9 droplets (droplet separation=35 μm) of 0.01 mM SoF (in H 2 O/glycerol, 1:1 v/v) was first patterned on a SiO 2 surface at DT 1 =0.001 s at room temperature under a RH of 60%. Femtolitre volumes of an H 2 O/glycerol (1:1) mixture were then delivered into the pre-patterned SoF droplets using a second microfluidic pen at DT 2 =0.001, 0.1, 0.5, 1.5, 2, 4, 6 and 8 s, starting from the second row. To evaluate the cross-contamination effect, an array of 1 × 8 droplets (droplet separation=35 μm) of 0.03 mM SoF (in H 2 O/glycerol, 1:1 v/v) was first patterned on a SiO 2 surface at DT 1 =0.001 s at room temperature under a RH of 45%. Then, femtolitre volumes of an H 2 O/glycerol (1:1) mixture were delivered into the pre-patterned SoF droplets using a second microfluidic pen at DT 2 =0.001, 0.01, 0.1, 1, 3, 5, 8 and 10 s. In this case, after each one of these eight deliveries, eight consecutive droplets (droplet separation=35 μm) of the H 2 O/glycerol (1:1) mixture were patterned at a DT=2 s. An SoF/Nile Blue mixture droplet array was fabricated by first patterning an array of 10 × 6 droplets (droplet separation=28 μm) of 0.01 M SoF (in H 2 O/glycerol, 1:1 v/v) on a SiO 2 surface at DT 1 =0.01 s at room temperature under a RH of 52%. Femtolitre volumes of 0.014 mM Nile Blue (in H 2 O/glycerol, 1:1 v/v) were then delivered into the pre-patterned droplets using a second microfluidic pen at DT 2 =0.001, 0.01, 0.1, 0.5, 2, 4, 8 and 10 s. MPL-assisted femtolitre reactions In a typical experiment, an array of droplets of a solution containing a reagent (R 1 ) was first patterned onto a SiO 2 surface at a certain DT 1 . Then, femtolitre volumes of a second solution containing another reagent (R 2 ) were delivered into the pre-patterned droplets using another microfluidic pen at an optimized DT 2 . This two-step process was performed at a certain RH. Unless otherwise noted, all resulting mixture droplets were then kept at RT under the same RH for a certain time ( t ) in order to conduct the intended reactions. Following this protocol, optimal reaction conditions were studied for the acid/base reaction and the enzymatic recognition reaction, as well as for the synthesis of HKUST-1, PBAs and metal-peptide coordination networks. The conditions used to perform these femtolitre reactions were: Acid-base reaction. R 1 : Fluorescein acid [2 mM, DMSO/glycerol (7:3)]; DT 1 : 0.001 s; 11 × 11 droplet array (droplet distance=25 μm); R 2 : KOH [0.34 M, H 2 O/glycerol (7:3)]; DT 2 : 0.1 s; RH: 50%; t : 1 min. Enzymatic recognition reaction. R 1 : BBTP [14 mM, AttoPhos buffer—Promega AttoPhos AP Fluorescent Substrate System, Technical Bulletin. http://www.promega.com , (2.4 M DEA, 0.057 mM MgCl 2 , 0.005% NaN 3 )]; DT 1 : 0.5 s; 10 × 10 droplet array (droplet distance=30 μm); R 2 : AP [1 unit 6 μl −1 (1 unit: amount of enzyme required to catalyse the hydrolysis of 1 μmol of 4-nitrophenyl phosphate per minute at 37 °C in 1 M DEA, 10.9 mM 4-nitrophenyl phosphate and 0.5 mM MgCl 2 (pH=9.8))]; DT 2 : 0.5 s; RH: 75%; t : 15 min. at 37 °C. HKUST-1 synthesis. R 1 : Cu(NO 3 ) 2· 2.5H 2 O [2.5 M, DMSO]; DT 1 : 0.001 s; 30 × 30 droplet array (droplet distance=20 μm); R 2 : Trimesic acid [1 M, DMSO/glycerol (8.5:1.5)]; DT 2 : 0.1 s; RH: 50%; t : 4 h. Combinatorial PBA synthesis. R 1 : K 3 Co(CN) 6 [0.1 M, H 2 O/glycerol (7.5:2.5)]; DT 1 : 1 s; 4 × 4 droplet array (droplet distance=20 μm); R 2 : M(NO 3 ) x ·yH 2 O [M=Mn(II) (0.18 M), Cd(II) (0.18 M), Zn(II) (0.18 M) and Ag(I) (0.36 M), H 2 O/glycerol (7.5:2.5)]; DT 2 : 0.5 s; RH: 50%; t : 0.5 h. Screening the formation/crystallization of metal-peptide networks. R 1 : GH [1 M, H 2 O]; DT 1 : 1 s; 3 × 7 droplet array (droplet distance=30 μm); R 2 : M(CH 3 COO) x ·y(H 2 O) (where M=Mn(II), Cd(II), Cu(II), Cr(III), Zn(II), Ni(II) and Co(II), 0.3 M, H 2 O:diethyleneglycol (7:3)); DT 2 : 0.01, 0.1 and 0.2 s; RH: 85%; t : 0.5 h. Array characterization SoF and mixture (SoF/H 2 O-glycerol and SoF/Nile Blue) droplet arrays were characterized by confocal fluorescence microscopy (LEICA TCS SP5). Stacks comprising 30 fluorescence microscopy image slices ( λ exc =488 nm; λ em =500–575 nm for SoF and λ exc =633 nm; λ em =600–785 nm for Nile Blue) at different heights (Δz=0.42 μm) were collected for each array. Confocal microscopy images were then used to determine the average droplet diameter ( d 1 and d 2 ), and therefore, the estimated average volumes of each droplet series, as further described in Supplementary Methods , Supplementary Figs S11,S12 and Supplementary Tables S6, S7 . Moreover, the same images were used to determine the average of the fluorescence mean intensity ( I / A ; defined as the sum of the intensities of all fluorescent pixels in a droplet divided by its area) for each droplet series, as detailed in Supplementary Methods . The data were analysed using ImageJ software. Importantly, d 1 and d 2 values determined from confocal microscope images were in full agreement with those determined from optical microscopy images. Acid-base and enzymatic recognition reactions, both involving fluorescent compounds, were followed by fluorescence optical microscopy (Zeiss Axio Observer Z-1). FESEM (Zeiss Merlin) and Energy Dispersive X-Ray (Oxford INCA X-Max) analysis were used to study the formation of the different MOF crystals. To confirm the formation of the desired PBA phases, electron diffraction analysis (Hitachi H-7000) was also performed on each one of the sixteen individual crystalline islands of the multiplexed array. Bulk reactions between metal salts and the dipeptide GH A quantity of 0.35 ml of an aqueous solution of 0.3 M M(CH 3 COO) x ·y(H 2 O) (where M=Cr(III), Mn(II), Co(II), Ni(II), Cu(II), Zn(II) and Cd(II)) was added into 2 ml of an aqueous solution of GH (1 mmol) in a 5-ml glass vial. The resulting mixtures were left standing at RT or heated at 90 °C for 2 h. Under the studied conditions, only the reactions (both at RT and 90 °C) between GH and Cu(CH 3 COO) 2 ·H 2 O or Ni(CH 3 COO) 2 ·4H 2 O afforded crystals suitable for single crystal analysis: dark blue (79% yield) and blue (62% yield), respectively (see Supplementary Tables S1–S5 ). Their phase purity was confirmed by XRPD (X’Pert PRO MPD diffractometer; Panalytical), IR (Tensor 27 FTIR spectrophotometer equipped with a Golden Gate diamond ATR cell; Bruker) and elemental analysis (see Supplementary Fig. S10 ). Interestingly, no formation of solid was observed in any of the reactions with the other metal ions, even after 1 week left standing at room temperature. Accession codes: The X-ray crystallographic coordinates for [Ni(GH) 2 ]·7H 2 O and [Cu(GH)(H 2 O)]·H 2 O reported in this Article have been deposited at the Cambridge Crystallographic Data Centre (CCDC), under deposition numbers CCDC 912266 and 912870, respectively. These data can be obtained free of charge from The Cambridge Crystallographic Data Centre via http://www.ccdc.cam.ac.uk/data_request/cif . How to cite this article: Carbonell, C. et al . Femtolitre Chemistry assisted by microfluidic pen lithography. Nat. Commun . 4:2173 doi: 10.1038/ncomms3173 (2013).